Phosphorylation of LKB1/Par-4 establishes Schwann cell polarity to initiate and control myelin extent The Schwann cell (SC)–axon interface represents a membrane specialization that integrates axonal signals to coordinate cytoskeletal dynamics resulting in myelination. Here we show that LKB1/Par-4 is asymmetrically localized to the SC–axon interface and co-localizes with the polarity protein Par-3. Using purified SCs and myelinating cocultures, we demonstrate that localization is dependent on the phosphorylation of LKB1 at serine-431. SC-specific deletion of LKB1 significantly attenuates developmental myelination, delaying the initiation and altering the myelin extent into adulthood, resulting in a 30% reduction in the conduction velocity along the adult sciatic nerves. Phosphorylation of LKB1 by protein kinase A is essential to establish the asymmetric localization of LKB1 and Par-3 and rescues the delay in myelination observed in the SC-specific knockout of LKB1. Our findings suggest that SC polarity may coordinate multiple signalling complexes that couple SC–axon contact to the redistribution of specific membrane components necessary to initiate and control myelin extent. Cell polarity is critical for various cellular processes including establishing the anteroposterior axis, generating distinct membrane specializations (apical and basal polarity), as well as asymmetric cell division and axon specification. Essentially, cell polarity plays fundamental roles to help organize and integrate complex molecular signals for cells to function properly and make decisions concerning fate and differentiation. One such group of factors, the partitioning defective (Par) proteins, is essential in mediating cell polarity through the formation of a molecular complex [1] , [2] . While the Par proteins were first identified in Caenorhabditis elegans [3] , they are remarkably conserved across various model organisms and cell types, implicating these proteins in a unique intrinsic programme that directs specified function in highly dynamic environments. The role of the Par complex in establishing cellular asymmetry is largely conserved in various cellular processes. However, the precise mechanisms may differ based on the cell-context specificity for adaptor proteins and the specific activation of downstream signalling pathways. Since the tumour suppressor protein LKB1/Par-4 mutations are epistatic to other Par protein functions, we propose that LKB1 may be the central regulator of cellular asymmetry in the Schwann cell (SC) [4] , [5] . Underlying this rationale are two specific findings: (1) the discovery for the role of Par-3 in the formation of a unique membrane specialization in the SC, similar to that observed in the apical polarity of epithelial cells [6] , [7] , [8] , [9] , [10] , and (2) the polarity proteins Pals1 and Dlg can modulate the extent of the myelin sheath (wraps of myelin) formed by SCs [11] , [12] . While much has been learned concerning the mechanisms and molecules responsible for the maintenance and stabilization of cell polarity, relatively little is known about the extrinsic cues that initiate asymmetry. In Fig. 1a , we illustrate the conservation and multifaceted roles for the Par polarity proteins during SC development that may facilitate the integration of multiple signalling pathways. The Par complex is asymmetrically localized to the site of the SC–axon interface [8] , [13] and may be recruited by various adhesion molecules, such as N-cadherin, Necl4 and/or the integrins [7] , [13] , [14] , [15] , [16] , as well as growth factor receptors [6] , [8] . In addition, the Par complex may reciprocally recruit growth factor receptors and/or adhesion molecules to initiate localized signalling cascades. The Par proteins can activate the Rho family of small GTPases to alter actin dynamics, important for the ensheathment and sorting of individual axons [17] , [18] , [19] , [20] . It is well established that the Par proteins can interact with various adaptor-like proteins that associate with and/or control the orientation and positioning of microtubules, essential for directed elongation and membrane spreading [21] , [22] , [23] , [24] , [25] , [26] , [27] , [28] , [29] , [30] , [31] , [32] . Finally, the Par complex can activate signalling pathways to influence cytoskeletal rearrangement as well as gene expression to promote the initiation and extent of myelination [11] , [12] , [33] , [34] , [35] , [36] , [37] , [38] , [39] , [40] , [41] ( Fig. 1a ). To date, six Par genes have been cloned and characterized, and Par-1 and Par-4 (also known as LKB1) are the only family members that encode serine-threonine kinases. As a multitude of extrinsic signals have been previously identified to converge on LKB1, combined with the fact that LKB1 can activate Par-1 via phosphorylation, we hypothesize that LKB1 may act as a central regulator to establish cellular asymmetry in the SC [1] , [4] , [42] . 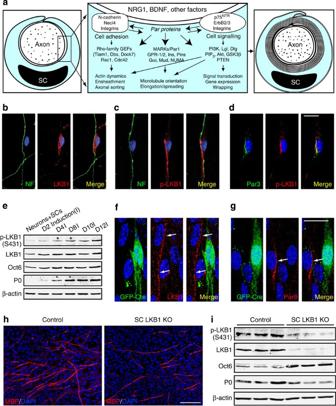Figure 1: The localization of LKB1 is essential for proper SC myelination. (a) A schematic illustration of the possible conservation and multifaceted roles for the Par polarity proteins during SC development and myelination. (b) Immunostaining of LKB1 (red) in purified SC-DRG cocultures illustrates that LKB1 is diffusely localized and enriched at SC–axon interface. Immunostaining of neurofilament illustrates the position of the neuronal axon (green). (c) Phosphorylated LKB1 (red) at ser-431 is asymmetrically localized to the SC–axon interface. (d) Phosphorylated LKB1 (red) co-localizes with Par-3 (green) at the SC–axon interface. The cell nuclei are detected by DAPI (blue). Scale bars=10 μm. (e) Western blot analysis of SC-DRG cocultures before and after induction of myelination by addition of ascorbic acid (denoted by the I). Western blots were probed with antibodies to phosphorylated ser-431 LKB1, LKB1, Oct-6 (a transcription factor expressed by premyelinating SCs) and the myelin protein P0. β-actin serves as a loading control. The asterisks indicate the concomitant expression of phosphorylated ser-431 with the myelin protein P0. (f) Floxed-LKB1 SC-DRG cocultures were established and SCs were transduced with a retrovirus to express Cre-recombinase and GFP (green). LKB1 immunostaining illustrates the knockdown of LKB1 expression in the transduced SCs. Arrows indicate the asymmetric localization of LKB1 in uninfected SCs. (g) Deletion of LKB1 in SCs disrupts the localization of Par-3 to the SC–axon interface. The arrow indicates the asymmetric localization of Par-3 (red) in the uninfected SC. The nuclei are detected with DAPI (blue). Scale bars=10 μm. (h) SC-DRG cocultures were established from crossing the floxed-LKB1 mice with the CNP-Cre mice and induced to myelinate for 10 days. Myelin internodes are identified with MBP staining (red) and nuclei are detected with DAPI (blue). Scale bar=100 μm. (i) Western blots from the SC-specific LKB1 knockout cocultures were probed with phos-ser-431 LKB1, LKB1, Oct-6 and the myelin protein P0. Representative western blots are displayed and all results were obtained from a minimum of three independent experiments (n=3). Figure 1: The localization of LKB1 is essential for proper SC myelination. ( a ) A schematic illustration of the possible conservation and multifaceted roles for the Par polarity proteins during SC development and myelination. ( b ) Immunostaining of LKB1 (red) in purified SC-DRG cocultures illustrates that LKB1 is diffusely localized and enriched at SC–axon interface. Immunostaining of neurofilament illustrates the position of the neuronal axon (green). ( c ) Phosphorylated LKB1 (red) at ser-431 is asymmetrically localized to the SC–axon interface. ( d ) Phosphorylated LKB1 (red) co-localizes with Par-3 (green) at the SC–axon interface. The cell nuclei are detected by DAPI (blue). Scale bars=10 μm. ( e ) Western blot analysis of SC-DRG cocultures before and after induction of myelination by addition of ascorbic acid (denoted by the I). Western blots were probed with antibodies to phosphorylated ser-431 LKB1, LKB1, Oct-6 (a transcription factor expressed by premyelinating SCs) and the myelin protein P0. β-actin serves as a loading control. The asterisks indicate the concomitant expression of phosphorylated ser-431 with the myelin protein P0. ( f ) Floxed-LKB1 SC-DRG cocultures were established and SCs were transduced with a retrovirus to express Cre-recombinase and GFP (green). LKB1 immunostaining illustrates the knockdown of LKB1 expression in the transduced SCs. Arrows indicate the asymmetric localization of LKB1 in uninfected SCs. ( g ) Deletion of LKB1 in SCs disrupts the localization of Par-3 to the SC–axon interface. The arrow indicates the asymmetric localization of Par-3 (red) in the uninfected SC. The nuclei are detected with DAPI (blue). Scale bars=10 μm. ( h ) SC-DRG cocultures were established from crossing the floxed-LKB1 mice with the CNP-Cre mice and induced to myelinate for 10 days. Myelin internodes are identified with MBP staining (red) and nuclei are detected with DAPI (blue). Scale bar=100 μm. ( i ) Western blots from the SC-specific LKB1 knockout cocultures were probed with phos-ser-431 LKB1, LKB1, Oct-6 and the myelin protein P0. Representative western blots are displayed and all results were obtained from a minimum of three independent experiments ( n =3). Full size image Here we demonstrate that LKB1 is asymmetrically localized to the SC–axon interface and co-localizes with the polarity protein Par-3. We find that the localization of LKB1 is dependent on phosphorylation at ser-431 and correlates with the expression of myelin-specific proteins. By generating a SC-specific knockout of LKB1, the asymmetric localization of Par-3 is disrupted and developmental myelination is significantly attenuated without altering SC proliferation or alignment. We demonstrate that the cAMP-dependent phosphorylation of LKB1 in SCs by PKA is necessary to establish the asymmetric localization of LKB1 and Par-3 and is capable of rescuing the hypomyelination phenotype observed in the SC-specific deletion of LKB1. Together, these findings illustrate the fascinating redundancy and conservation of the molecular mechanisms involved in the establishment of cellular asymmetry and provide valuable insight into the mechanisms surrounding the initiation of membrane wrapping and extent of the myelin sheath. Asymmetric localization of LKB1 to the SC–axon interface What are the initial steps that break symmetry within a cell and what insight does this understanding provide for SC myelination? Evidence for the role of LKB1 in the generation of cellular asymmetry in the SC requires two key components: (1) the localization of LKB1 should most likely be polarized (asymmetrically distributed) and (2) the localization of LKB1 should be intimately associated with activation. LKB1 contains a number of residues that are either autophosphorylated or phosphorylated by upstream kinases (ser-31, ser-325, thr-366 and ser-431). These sites are highly conserved in drosophila, xenopus and mammalian cells [4] , [42] . However, only ser-431 alters the cellular localization of LKB1 (refs 43 , 44 ). Therefore, we examined the expression and phosphorylation of LKB1 during development in purified SC-DRG cocultures [13] . Consistent with our hypothesis, the localization of LKB1 is dependent on the phosphorylation of ser-431. While LKB1 is enriched at the SC–axon interface, it is diffusely localized throughout the SC body and SC processes ( Fig. 1b ), phosphorylated LKB1 is asymmetrically localized to the SC–axon interface ( Fig. 1c ) and co-localizes with Par-3 ( Fig. 1d ), similar to our previous observations with N-cadherin and β-catenin [8] , [13] . In addition, phosphorylation at ser-431 of LKB1 correlates with the induction of SC myelination by the addition of ascorbic acid and precedes the expression of the myelin protein P0 ( Fig. 1e , asterisks). To examine the potential role of LKB1 during SC development in vitro , we initially established SC-DRG cocultures from the floxed-LKB1 mice and transduced Cre-recombinase with green fluorescent protein (GFP) into SCs using retrovirus. As the retroviral vectors infect only actively dividing cells, this system ensures that SCs are specifically infected, whereas the DRG neurons remain uninfected. Knockdown of the LKB1 was confirmed in the SCs by immunostaining for LKB1 ( Fig. 1f ). In addition, deletion of LKB1 disrupted the asymmetric localization of Par-3, suggesting that LKB1 is necessary for the redistribution of Par-3 to the SC–axon interface ( Fig. 1g ). As proliferation and alignment of SCs in the cocultures are unaffected by deletion of LKB1, we sought to examine the role of LKB1 on the initiation of myelination. Therefore, we generated the SC-specific deletion of LKB1 by crossing the floxed-LKB1 mice with the CNP-Cre mice. In these mice, the cre-recombinase is under the control of the CNP gene regulatory sequences and is expressed in SCs from E12 (ref. 17 ). Upon establishing the SC-DRG cocultures, we quickly observed a significant decrease in the number of myelin internodes from the SC-specific knockout (KO) cultures as compared with the wild-type (WT) controls ( Fig. 1h ). Western blot analyses illustrate the deletion of LKB1 from the SC-DRG cocultures ( Fig. 1i ). While the expression of the myelin protein P0 is significantly attenuated in the knockout SC-DRG cocultures, we detect a concomitant increase in the expression of the transcription factor Oct-6, suggesting that the LKB1 KO SCs are held in a more immature state ( Fig. 1i ). SC-specific knockout of LKB1 attenuates myelination To investigate the role of LKB1 during the development of the peripheral nervous system in vivo , we analysed WT and the LKB1 SC-specific KO mice at different times during postnatal development. While the mice are slightly smaller than littermate controls ( Fig. 2a ), the sciatic nerve at 7 days postnatal displays a severe hypomyelination phenotype, as the nerve is translucent and significantly thinner ( Fig. 2b ). To confirm that LKB1 is indeed deleted, we immunostained sciatic nerve sections for LKB1 and observed a considerable decrease in LKB1 expression in the SCs as compared with littermate controls ( Fig. 2d ). Sciatic nerves from WT littermates and the LKB1 SC-specific KO mice at postnatal day 7, 14 and 60 were collected, stained with luxol fast blue and analysed using light microscopy. At postnatal days 7 and 14, it is evident that the initiation of myelination is significantly delayed and that myelin extent is diminished ( Fig. 2c ). However, after waiting for an additional 2 months postnatal, the LKB1 SC-specific KO mice display many more myelinated axons; however, the myelin extent appears to remain decreased as compared with littermate controls ( Fig. 2c ), suggesting that both initiation and myelin extent are altered. These observations are consistent with the hypothesis that cell polarity may regulate the initiation of myelination via cytoskeletal rearrangement and, in addition, control the myelin extent by modulating signal transduction pathways and gene expression ( Fig. 1a ). Western blot analyses of the sciatic nerves from three littermate WT and three SC-specific KO mice at postnatal day 14 were performed ( Fig. 2e ). Similar to immunostaining, LKB1 expression is clearly diminished in the SC-specific KO nerves. Oct-6 expression is elevated in the KO nerves and P0 is greatly attenuated. These findings are consistent with our in vitro results and suggest an important role for LKB1 in the maturation of the SC and the initiation of myelination. 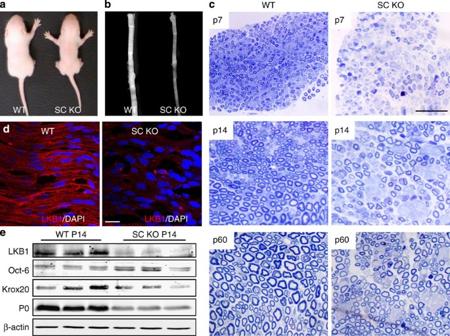Figure 2: SC-specific knockout of LKB1 attenuates myelination during development. (a) SC-specific deletion of LKB1 was accomplished by crossing the floxed-LKB1 mice with the CNP-Cre mice. (b) Sciatic nerves from a WT littermate and the SC-specific LKB1 KO mice. (c) Time course of sciatic nerve myelination in WT littermates and SC-specific LKB1 KOs at 7, 14 and 60 days postnatal with Luxol Fast Blue staining. Scale bar=10 μm. (d) Immunostaining for LKB1 (red) from the sciatic nerves in the WT littermate and the SC-specific LKB1 KO mice. Scale bar=10 μm. (e) Western blots of WT littermates and SC-specific LKB1 KO nerves at 14 days postnatal were probed with antibodies to LKB1, Oct-6, Krox20 and the myelin protein P0. β-actin serves as a loading control. Representative western blots and sciatic nerves are displayed from three knockout and three WT littermates. Figure 2: SC-specific knockout of LKB1 attenuates myelination during development. ( a ) SC-specific deletion of LKB1 was accomplished by crossing the floxed-LKB1 mice with the CNP-Cre mice. ( b ) Sciatic nerves from a WT littermate and the SC-specific LKB1 KO mice. ( c ) Time course of sciatic nerve myelination in WT littermates and SC-specific LKB1 KOs at 7, 14 and 60 days postnatal with Luxol Fast Blue staining. Scale bar=10 μm. ( d ) Immunostaining for LKB1 (red) from the sciatic nerves in the WT littermate and the SC-specific LKB1 KO mice. Scale bar=10 μm. ( e ) Western blots of WT littermates and SC-specific LKB1 KO nerves at 14 days postnatal were probed with antibodies to LKB1, Oct-6, Krox20 and the myelin protein P0. β-actin serves as a loading control. Representative western blots and sciatic nerves are displayed from three knockout and three WT littermates. Full size image After the second postnatal week, nerve sections were immunostained for Krox20, a transcription factor expressed specifically in myelinating SCs, as well as Oct-6 and Sox2, transcription factors expressed in premyelinating and non-myelinating SCs ( Fig. 3a–e ). Krox20 expression is robust in the myelinating SCs of the WT nerves and is significantly attenuated in the SC-specific KO nerves ( Fig. 3e ). Oct-6 and Sox2 expression levels are elevated in the SC-specific KO nerves as compared with WT controls ( Fig. 3e ). The quantification of the p14 nerves suggests that the LKB1 KO SCs are held in an immature state, resulting in the delayed expression of Krox20. It is important to note that the total number of SCs is unchanged along the sciatic nerves from the WT and SC-specific KO mice. Sciatic nerves were also immunostained with S100β (green) and myelin basic protein (MBP; red) to examine potential effects on SC numbers and myelination ( Fig. 3g–j ). Myelin internodes are greatly diminished in the SC-specific KO nerves as compared with WT controls ( Fig. 3f–h ), consistent with the luxol fast blue staining ( Fig. 2c ). In addition, the number of SCs is essentially unchanged upon quantification of S100β immunostaining ( Fig. 3f ). Upon examination of SCs stained with S100β, it is evident that the SCs are elongating along the axons and similar in morphology to the WT SCs ( Fig. 3i,j ). Electron micrographs from the sciatic nerves were also examined and found to be consistent with the previous findings, that deletion of LKB1 in SCs significantly attenuates developmental myelination, delaying the initiation and altering the myelin extent into adulthood ( Fig. 4a ). Examination of micrographs at postnatal day 14 resulted in the identification of numerous unmyelinated axons that were not yet sorted by individual SCs ( Fig. 4b ), similar to observations in the Rac1 knockout mice [17] , [18] . Quantification of the number of myelinated axons from the sciatic nerves displays a significant decrease at postnatal days 7 and 14; however, this difference is no longer apparent at 2 months of age ( Fig. 4c ). From both light and electron microscopy, it is evident that myelin extent is greatly diminished in the LKB1 SC-specific KO nerves even at 2 months postnatal. This is clearly evident when comparing the myelin from similar-sized axons from WT and LKB1 SC-specific KO nerves ( Fig. 4d ). G-ratios display an overall increase in the SC-specific KO nerves, indicative of a decrease in the extent of myelin thickness at day 60 postnatal. These findings clearly indicate that the myelin extent from the SC-specific KO nerves remains thinner even in adulthood and does not simply represent a delay in onset of myelination ( Fig. 4e , Supplementary Fig. 1 ). Together, these results suggest that LKB1 in SCs is an essential regulator for the timely initiation of myelination and controls the extent of myelination into adulthood. 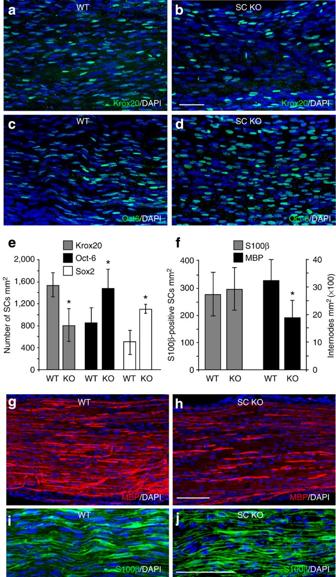Figure 3: Knockout of LKB1 delays the maturation of SCs and myelination. (a,b) Immunostaining for Krox20 (green) illustrates the number of promyelinating and myelinating SCs along the sciatic nerve of a WT littermate and the SC-specific LKB1 KO at 14 days postnatal. (c,d) Immunostaining for Oct-6 (green) illustrates the number of premyelinating SCs. Scale bar=100 μm. (e,f) Quantification of the number of Oct-6−, Krox20−, Sox2−, S100β-positive SCs per mm2and number of MBP-positive myelin internodes per mm2in the WT littermate and the SC-specific LKB1 KO sciatic nerves at 14 days postnatal. Error bars represent s.d. Asterisks represent significance based on Student’st-test as compared with the WT control (P<0.004). (g,h) Immunostaining for MBP (red) illustrates the myelin internodes in the sciatic nerve of a WT littermate and the SC-specific LKB1 KO at 14 days postnatal. Scale bar=100 μm. (i,j) S100β (green) illustrates the number of SCs along the sciatic nerve of a WT littermate and the SC-specific LKB1 KO at 14 days postnatal. Scale bar=100 μm. Nuclei are detected by DAPI (blue). Results are obtained from three knockout and three WT littermates. Figure 3: Knockout of LKB1 delays the maturation of SCs and myelination. ( a , b ) Immunostaining for Krox20 (green) illustrates the number of promyelinating and myelinating SCs along the sciatic nerve of a WT littermate and the SC-specific LKB1 KO at 14 days postnatal. ( c , d ) Immunostaining for Oct-6 (green) illustrates the number of premyelinating SCs. Scale bar=100 μm. ( e , f ) Quantification of the number of Oct-6−, Krox20−, Sox2−, S100β-positive SCs per mm 2 and number of MBP-positive myelin internodes per mm 2 in the WT littermate and the SC-specific LKB1 KO sciatic nerves at 14 days postnatal. Error bars represent s.d. Asterisks represent significance based on Student’s t -test as compared with the WT control ( P <0.004). ( g , h ) Immunostaining for MBP (red) illustrates the myelin internodes in the sciatic nerve of a WT littermate and the SC-specific LKB1 KO at 14 days postnatal. Scale bar=100 μm. ( i , j ) S100β (green) illustrates the number of SCs along the sciatic nerve of a WT littermate and the SC-specific LKB1 KO at 14 days postnatal. Scale bar=100 μm. Nuclei are detected by DAPI (blue). Results are obtained from three knockout and three WT littermates. 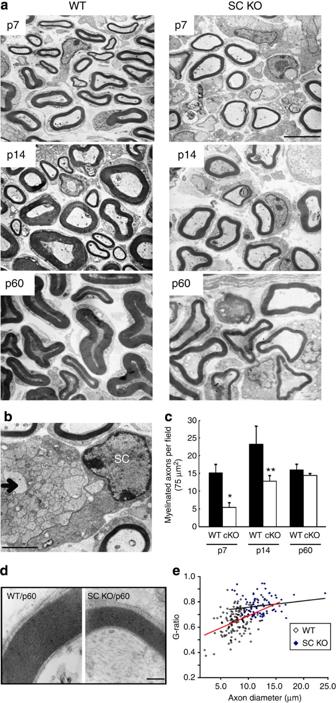Figure 4: Knockout of LKB1 delays the initiation and alters myelin extent. (a) The sciatic nerves from SC-specific LKB1 KO and WT littermate mice at postnatal days 7, 14 and 60 were isolated and processed for electron microscopy. Scale bar=2.5 μm. (b) Electron micrograph of a sciatic nerve from SC-specific LKB1 KO mouse at 14 days postnatal illustrating a SC nucleus and unmyelinated axons (arrow). Scale bar=2.5 μm. (c) Quantification of the number of myelinated axons per 75 μm2in the WT littermate (black bars) and the SC-specific LKB1 KO (white bars) at 7, 14 and 60 days postnatal. Error bars represent s.d. Asterisk represents significance based on Student’st-test as compared with the WT control (*P<0.05, **P<0.01). (d) High-resolution electron micrographs of myelin from WT littermate and the SC-specific LKB1 KO mice at 60 days postnatal. Scale bar=200 nm. (e) Determination of myelin sheath thickness by G-ratio quantification from sciatic nerves isolated from three WT and three SC-specific LKB1 KO mice. Full size image Figure 4: Knockout of LKB1 delays the initiation and alters myelin extent. ( a ) The sciatic nerves from SC-specific LKB1 KO and WT littermate mice at postnatal days 7, 14 and 60 were isolated and processed for electron microscopy. Scale bar=2.5 μm. ( b ) Electron micrograph of a sciatic nerve from SC-specific LKB1 KO mouse at 14 days postnatal illustrating a SC nucleus and unmyelinated axons (arrow). Scale bar=2.5 μm. ( c ) Quantification of the number of myelinated axons per 75 μm 2 in the WT littermate (black bars) and the SC-specific LKB1 KO (white bars) at 7, 14 and 60 days postnatal. Error bars represent s.d. Asterisk represents significance based on Student’s t -test as compared with the WT control (* P <0.05, ** P <0.01). ( d ) High-resolution electron micrographs of myelin from WT littermate and the SC-specific LKB1 KO mice at 60 days postnatal. Scale bar=200 nm. ( e ) Determination of myelin sheath thickness by G-ratio quantification from sciatic nerves isolated from three WT and three SC-specific LKB1 KO mice. Full size image Knockout of LKB1 attenuates conduction velocity As deletion of LKB1 from SCs results in significantly thinner myelin extent, we hypothesize that thinner myelin would result in increased membrane capacitance and lead to functional deficits reflected by delayed conduction velocity measurements. Therefore, we measured compound action potentials (CAPs) in isolated sciatic nerves. Consistent with our hypothesis, the SC-specific KO sciatic nerves displayed a 30.8% reduction in the conduction velocity, as compared with WT littermates (WT: 11.8±0.92 m s −1 versus cKO: 8.2±0.66 m s −1 ; Fig. 5a,b ). The threshold stimulus for maximal CAP responses was measured and found to be similar between both genotypes (WT: 0.53±0.087 mA versus cKO: 0.56±0.075 mA; Fig. 5c ). In addition, we performed paired stimulation experiments to examine whether the SC-specific knockout of LKB1 alters the refractory period of the nerves. The refractory periods between genotypes were not significantly altered ( Fig. 5d,e ). These findings suggest that the increase in membrane capacitance as a result of the thinner myelin in the KO mice results in the attenuation in the propagation of the action potential. Together, these findings demonstrate that the long-term consequence of decreased myelin extent can be detected by electrophysiological analysis and may result in functional deficits in physiology and behaviour of the SC-specific LKB1 KO mice. 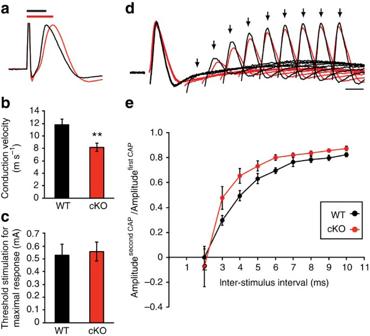Figure 5: Knockout of LKB1 attenuates the conduction velocity. (a) Representative-overlaid traces of CAP recordings from isolated sciatic nerves illustrating the difference in latency between stimulation and CAP peak in WT (black trace/bar) and SC-specific LKB1 knockout nerves (red trace/bar). Traces are scaled to match CAP amplitude for latency comparison. (b) Conduction velocity of WT and SC-specific LKB1 knockout nerves (**P<0.01). (c) Threshold stimulation of current for evoking maximal CAP responses. (a–c)n=7 nerves, four mice from each genotype. (d) Representative overlaid traces of CAP recordings from paired stimulation experiments illustrating the recovery of amplitude in the second CAP (black arrows) from the refractory period with increasing interstimulus interval. Traces are scaled and aligned to match amplitude and timing of the first CAP. (e) The ratio of the amplitude of the second CAP over that of the first in paired stimulation experiments. Displayed traces are the average of 10 individual recordings. Stimulus artifacts are truncated for clarity. (d,e)n=4 nerves, three mice from WT,n=5 nerves, three mice from LKB1 cKO. The red line inaand the black scale bar indrepresent 1 ms. Figure 5: Knockout of LKB1 attenuates the conduction velocity. ( a ) Representative-overlaid traces of CAP recordings from isolated sciatic nerves illustrating the difference in latency between stimulation and CAP peak in WT (black trace/bar) and SC-specific LKB1 knockout nerves (red trace/bar). Traces are scaled to match CAP amplitude for latency comparison. ( b ) Conduction velocity of WT and SC-specific LKB1 knockout nerves (** P <0.01). ( c ) Threshold stimulation of current for evoking maximal CAP responses. ( a – c ) n =7 nerves, four mice from each genotype. ( d ) Representative overlaid traces of CAP recordings from paired stimulation experiments illustrating the recovery of amplitude in the second CAP (black arrows) from the refractory period with increasing interstimulus interval. Traces are scaled and aligned to match amplitude and timing of the first CAP. ( e ) The ratio of the amplitude of the second CAP over that of the first in paired stimulation experiments. Displayed traces are the average of 10 individual recordings. Stimulus artifacts are truncated for clarity. ( d , e ) n =4 nerves, three mice from WT, n =5 nerves, three mice from LKB1 cKO. The red line in a and the black scale bar in d represent 1 ms. Full size image Phosphorylation of LKB1 by PKA regulates myelination Our data indicate that the asymmetric localization of LKB1 may be dependent on the phosphorylation of ser-431 of LKB1 ( Fig. 1c–e ). Analysis of the expression of phosphorylated ser-431 of LKB1 during normal sciatic nerve development indicates that phosphorylation precedes the expression of the myelin proteins P0 and MBP and correlates with the downregulation of Oct-6 ( Fig. 6a ; asterisks). In order to determine the upstream kinase involved in the phosphorylation of LKB1, we decided to examine the role of protein kinase A (PKA). Previous findings clearly demonstrate that ser-431 of LKB1 is an evolutionarily conserved PKA phosphorylation site across multiple species [4] , [42] , [45] , [46] . As PKA may be activated by cAMP and is essential for SC development [47] , [48] , [49] , we initially set out to determine whether phosphorylation of LKB1 is dependent on cAMP. SCs were purified and cultured in increasing concentrations (2–10 μM) of forskolin for 48 h to elevate cAMP, as well as the growth factors brain-derived neurotrophic factor (BDNF) or neureguilin-1 (NRG-1; Fig. 6b ). Phosphorylation of ser-431 of LKB1 was induced upon addition of forskolin at all concentrations tested as well as BDNF and NRG-1 ( Fig. 6b ). To confirm that PKA controls SC development and myelination via phosphorylation of LKB1, we expressed a dominant-negative (DN) form of PKA by targeting the alpha-1 catalytic subunit ( Fig. 6c ). Expression of the DN-PKA in SCs using a retroviral vector abolishes the expression and asymmetric localization of phosphorylated ser-431 of LKB1 in SCs ( Fig. 6d,e ). In addition, expression of the DN-PKA in SC-DRG cocultures significantly inhibits myelination by SCs, consistent with previous findings that suggest an essential role for PKA in SC myelination [47] ( Fig. 6f–i ). These results suggest that phosphorylation of LKB1 at ser-431 is dependent on cAMP/PKA signalling and function. 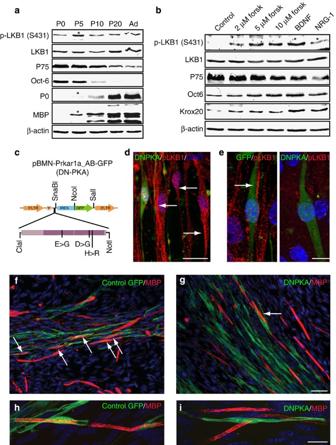Figure 6: Phosphorylation of LKB1 by PKA regulates localization and myelination. (a) Westerns blots of WT sciatic nerves at 0, 5, 10, 20 and 60 (ad) days postnatal were probed with antibodies to phospho-ser-431 of LKB1, LKB1, p75NTR, Oct-6 and the myelin proteins P0 and MBP. β-actin serves as a loading control. The asterisks indicate the concomitant expression of phosphorylated ser-431 with the myelin proteins P0 and MBP. (b) Purified rat SCs were isolated, cultured and treated with 2–10 μM forskolin, BDNF (10 ng ml−1) and NRG-1 (10 ng ml−1). Cultures were extracted for western blot analysis and samples were probed for phospho-ser-431 of LKB1, LKB1, p75NTR, Oct-6 and the transcription factor Krox20 (promyelinating SCs). β-actin serves as a loading control. (c) Illustration of the retroviral construct containing the DN PKA. (d,e) Purified SC-DRG cocultures were infected with the control or DN-PKA retrovirus. (d) On the basis of the construct design, GFP-positive SCs concomitantly express the DN-PKA and cultures were immunostained for phospho-LKB1 (red). (e) Control-infected SCs (left panel) and DN-PKA-infected SCs were immunostained for phospho-LKB1 (red). Arrows illustrate the asymmetric localization of the phospho-LKB1 in the uninfected SCs (d) and control-infected SCs (e). Scale bar=10 μm. (f,g) SC-DRG cocultures transduced with the control (f) and DN-PKA (g) retrovirus (green) were induced to myelinate for 10 days and immunostained for MBP (red). Scale bar=50 μm. (h,i) High-magnification images of control and DN-PKA-infected SCs (green) immunostained for MBP. Scale bar=10 μm. Cell nuclei are identified with DAPI (blue). All experiments were performed in triplicate and representative images are displayed. Figure 6: Phosphorylation of LKB1 by PKA regulates localization and myelination. ( a ) Westerns blots of WT sciatic nerves at 0, 5, 10, 20 and 60 (ad) days postnatal were probed with antibodies to phospho-ser-431 of LKB1, LKB1, p75 NTR , Oct-6 and the myelin proteins P0 and MBP. β-actin serves as a loading control. The asterisks indicate the concomitant expression of phosphorylated ser-431 with the myelin proteins P0 and MBP. ( b ) Purified rat SCs were isolated, cultured and treated with 2–10 μM forskolin, BDNF (10 ng ml −1 ) and NRG-1 (10 ng ml −1 ). Cultures were extracted for western blot analysis and samples were probed for phospho-ser-431 of LKB1, LKB1, p75 NTR , Oct-6 and the transcription factor Krox20 (promyelinating SCs). β-actin serves as a loading control. ( c ) Illustration of the retroviral construct containing the DN PKA. ( d , e ) Purified SC-DRG cocultures were infected with the control or DN-PKA retrovirus. ( d ) On the basis of the construct design, GFP-positive SCs concomitantly express the DN-PKA and cultures were immunostained for phospho-LKB1 (red). ( e ) Control-infected SCs (left panel) and DN-PKA-infected SCs were immunostained for phospho-LKB1 (red). Arrows illustrate the asymmetric localization of the phospho-LKB1 in the uninfected SCs ( d ) and control-infected SCs ( e ). Scale bar=10 μm. ( f , g ) SC-DRG cocultures transduced with the control ( f ) and DN-PKA ( g ) retrovirus (green) were induced to myelinate for 10 days and immunostained for MBP (red). Scale bar=50 μm. ( h , i ) High-magnification images of control and DN-PKA-infected SCs (green) immunostained for MBP. Scale bar=10 μm. Cell nuclei are identified with DAPI (blue). All experiments were performed in triplicate and representative images are displayed. Full size image Phosphorylation of LKB1 rescues myelination Finally, to determine whether phosphorylation of LKB1 is necessary and sufficient for SC function, we expressed WT LKB1 and the phosphorylation serine-431-alanine (S431A) mutant LKB1 into the LKB1 null SC background. SCs from the LKB1 SC-specific KO mice were cocultured with DRG neurons and transduced with either the full-length WT or S431A LKB1 ( Fig. 7a ). WT LKB1 correctly localizes to the SC–axon interface and is properly phosphorylated at ser-431, while the S431A mutant LKB1 is diffusely expressed and phosphorylation is essentially undetectable ( Fig. 7b,c ). In addition, WT LKB1 co-localizes with Par-3 at the SC–axon interface, while the S431A mutant abolishes the asymmetric localization of Par-3, suggesting that phosphorylation of LKB1 at ser-431 is essential for the redistribution of Par-3 ( Fig. 7d ). Western blot analysis of the cocultures demonstrates that forced expression of WT LKB1 in the null background is sufficient to rescue P0 expression and the concomitant downregulation of Oct-6 ( Fig. 7e,f ), suggesting that LKB1 is required for the maturation of the SC. Alternatively, forced expression of the S431A LKB1 does not rescue the expression of P0 or the downregulation of Oct-6, suggesting that phosphorylation of ser-431 of LKB1 is essential for the progression of premyelinating SCs into promyelinating SCs ( Fig. 7e,f ). SCs in a LKB1 null background were infected with WT, S431A and S431D LKB1 (phosphomimetic, Fig. 7g ) and were examined in cocultures. Quantification of the myelin internodes formed in the cocultures indicates that WT and S431D LKB1 rescue the hypomyelination phenotype by approximately threefold over the S431A mutant LKB1 ( Fig. 7h–k ). SC myelin internodes expressing the WT and S431D LKB1 are identified by the co-expression of GFP, while the S431A mutant LKB1 is rarely expressed in SCs actively making myelin internodes, albeit diminished in the LKB1 null background ( Fig. 7h–k ). These findings suggest that phosphorylation of LKB1 at S431 is essential to promote the timely initiation of myelination in vitro . However, to examine both necessity and sufficiency of phosphorylation of LKB1 by PKA during SC development, we co-transduced the DN-PKA construct and the S431D LKB1 into SCs in the LKB1 null background ( Fig. 7l ). Once again, the expression of the DN-PKA in SC-DRG cocultures significantly inhibits myelination by SCs. While the expression of the WT or S431D phosphomimetic LKB1 significantly rescues the myelination phenotype in the LKB1 null SCs ( Fig. 7m,n ), neither was sufficient to rescue myelination in the presence of the DN-PKA ( Fig. 7o ). These findings suggest that PKA function is dominant over LKB1 and that the additional function(s) of PKA contribute to the timely initiation of myelination, including but not limited to the phosphorylation of LKB1. 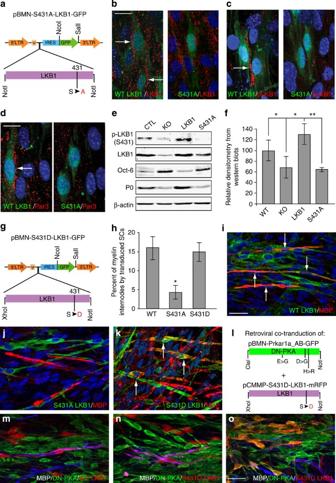Figure 7: Phosphorylation of LKB1 is essential to rescue the delay in myelination. (a) Illustration of the retroviral construct containing the serine-431–alanine LKB1 phosphorylation mutant. (b) SC-DRG cocultures were established from the SC-specific LKB1 knockout mice. SCs were infected with the WT or S431A LKB1 retrovirus and immunostained for LKB1 (red). Arrows illustrate the localization of LKB1 to the SC–axon interface. Scale bar=10 μm. (c) SCs infected with the WT or S431A LKB1 retrovirus were immunostained for phospho-Ser-431 LKB1 (red). Arrow illustrates the localization of phospho-ser-431 LKB1 to the SC–axon interface. (d) SCs infected with the WT or S431A LKB1 retrovirus were immunostained for Par-3 (red). Arrow illustrates the localization of Par-3 to the SC–axon interface. Scale bar=10 μm. (e) SCs infected with the WT or S431A LKB1 retrovirus were extracted and analysed with western blot analysis. Samples were probed with antibodies to phospho-ser-431 of LKB1, LKB1, Oct-6 and the myelin protein P0. β-actin serves as a loading control. (f) Quantification of the western blots was accomplished by measuring the relative densitometry. The asterisks represent significance based on Student’st-test as compared with the WT cultures (*P<0.05) or the WT-LKB1 rescue (**P<0.01). (g) Illustration of the retroviral construct containing the serine-431-aspartic acid LKB1 phosphomimetic. (h–k) SCs infected with the WT, S431A or S431D LKB1 retrovirus were induced to myelinate for 10 days. The cocultures were stained with MBP and the percent of myelin internodes formed by the infected SCs was quantified (h). The error bars represent s.d. and *P<0.05. (i,k) Arrows indicate transduced cells (green) forming myelin (MBP, red). (i) Scale bar=50 μm. (l) Illustration of the co-transduction of the retroviral constructs containing the DN-PKA and the S431D LKB1 phosphomimetic. (m–o) SCs co-transduced with the DN-PKA (green) and WT (m, red) or S431D LKB1 (n,o, red) retrovirus were induced to myelinate for 10 days. The cocultures were stained for MBP. Scale bar=50 μm. (o) Co-transduced SCs (yellow) were not observed to express MBP at anytime. All experiments were performed in triplicate and representative images are displayed. Figure 7: Phosphorylation of LKB1 is essential to rescue the delay in myelination. ( a ) Illustration of the retroviral construct containing the serine-431–alanine LKB1 phosphorylation mutant. ( b ) SC-DRG cocultures were established from the SC-specific LKB1 knockout mice. SCs were infected with the WT or S431A LKB1 retrovirus and immunostained for LKB1 (red). Arrows illustrate the localization of LKB1 to the SC–axon interface. Scale bar=10 μm. ( c ) SCs infected with the WT or S431A LKB1 retrovirus were immunostained for phospho-Ser-431 LKB1 (red). Arrow illustrates the localization of phospho-ser-431 LKB1 to the SC–axon interface. ( d ) SCs infected with the WT or S431A LKB1 retrovirus were immunostained for Par-3 (red). Arrow illustrates the localization of Par-3 to the SC–axon interface. Scale bar=10 μm. ( e ) SCs infected with the WT or S431A LKB1 retrovirus were extracted and analysed with western blot analysis. Samples were probed with antibodies to phospho-ser-431 of LKB1, LKB1, Oct-6 and the myelin protein P0. β-actin serves as a loading control. ( f ) Quantification of the western blots was accomplished by measuring the relative densitometry. The asterisks represent significance based on Student’s t -test as compared with the WT cultures (* P <0.05) or the WT-LKB1 rescue (** P <0.01). ( g ) Illustration of the retroviral construct containing the serine-431-aspartic acid LKB1 phosphomimetic. ( h – k ) SCs infected with the WT, S431A or S431D LKB1 retrovirus were induced to myelinate for 10 days. The cocultures were stained with MBP and the percent of myelin internodes formed by the infected SCs was quantified ( h ). The error bars represent s.d. and * P <0.05. ( i , k ) Arrows indicate transduced cells (green) forming myelin (MBP, red). ( i ) Scale bar=50 μm. ( l ) Illustration of the co-transduction of the retroviral constructs containing the DN-PKA and the S431D LKB1 phosphomimetic. ( m – o ) SCs co-transduced with the DN-PKA (green) and WT ( m , red) or S431D LKB1 ( n , o , red) retrovirus were induced to myelinate for 10 days. The cocultures were stained for MBP. Scale bar=50 μm. ( o ) Co-transduced SCs (yellow) were not observed to express MBP at anytime. All experiments were performed in triplicate and representative images are displayed. Full size image Myelination is a unique example of cell–cell interaction, whereby the SC wraps multiple layers of its own membrane around an axon to maximize the efficiency of the functioning neuron. How is this process initiated and how is myelination spatially and temporally regulated? Interestingly, there is remarkable redundancy in the function of Par proteins and various adhesion molecules that mediate numerous cellular processes. The Par proteins are undoubtedly the key players in mediating cell polarity, altering cytoskeletal dynamics, morphology and localizing signalling cascades essential for myelination. However, the lingering question is: how is SC polarity initially established? A requisite component for SC development and myelination is axonal contact and axon-derived signals, such as NRG-1 type III [35] , [36] . Herein, we find a paradoxical interaction, which links the intrinsic cellular mechanisms that establish cell polarity to extrinsic signals, and transduction of extrinsic signals to illicit specific function depends on the intrinsic nature of the cell. While there are still many questions remaining, our findings begin to illustrate how the intrinsic mechanism of SC polarity may transduce extrinsic signals into the initiation of myelination by the formation of a novel membrane specialization similar to the apical membrane domain of epithelial cells. We demonstrate that the polarity protein LKB1 may be the central regulator of cellular asymmetry in the SC to initiate myelination and control the proper extent. Our data illustrate that LKB1 is asymmetrically localized to the SC–axon interface and controls the redistribution of the polarity protein Par-3. The localization of LKB1 is dependent on phosphorylation at ser-431 by PKA and that this event is necessary to rescue the hypomyelination phenotype observed in the SC-specific deletion of LKB1. Our findings begin to couple the mechanisms surrounding the initiation of membrane wrapping with the proper extent of the myelin sheath. While these processes are thought to be mutually exclusive, the finding that Par-3 is essential for the proper initiation of myelination [6] , [7] , [8] , [9] , [10] , combined with data demonstrating that Pals1 and Dlg modulate the thickness of myelin sheath [11] , [12] , suggest that a single molecule, namely LKB1, may facilitate the integration of multiple signalling pathways. Previous findings concerning axon-derived NRG-1 type III and the activation of the PI3K/Akt/mTOR pathway [50] , [51] , [52] , [53] , [54] , [55] as important regulators of myelin extent suggest that initiation of cellular asymmetry may result in a convergence of pathways that result in myelination. In addition, sustained activation of ERK1/2 MAPK enhances myelin extent in SCs and oligodendrocytes [56] . It will be fascinating to examine the redundancy and conservation of the molecular mechanisms involved in the establishment of cellular asymmetry and the signalling pathways surrounding the initiation of membrane wrapping and extent of the myelin sheath. It is interesting to note that CNP-Cre mice also target oligodendrocyte precursor cells. Upon further examination, oligodendrocyte differentiation and myelination were essentially normal without delay in initiation or change in myelin extent ( Supplementary Fig. 2 ). The SC–axon interface represents a centralized position to provide orientation to the SC and allows it to transduce axonal signals into pathways that promote growth, trafficking and cytoskeletal rearrangement. While beyond the scope of this manuscript, we hope to one day elucidate the sequence of events and pathways that help to organize the construction and stabilization of this molecular scaffold at the SC–axon interface. Our findings provide us with a rare opportunity to begin to characterize this novel molecular scaffold, essential for the proper initiation and extent of myelination. Investigating the role of cell polarity during SC development should provide valuable insight into our understanding of the coordination of cytoskeletal dynamics, membrane trafficking and gene expression for the initiation, growth and maintenance of myelination. Generation of SC-specific LKB1 knockout mice and genotyping Mice were housed and maintained in the Laboratory Animal Resource Center at the University of California, San Francisco in accordance with all Institutional Animal Care and Use Committee requirements. CNP-Cre mice were a gift from (Dr Klaus Nave) and floxed-LKB1 mice were purchased from the Jackson Laboratory. Genomic DNA was isolated from mouse tails and standard PCR reactions were performed with the following primers: LKB1 Forward: 5′- ATCGGAATGTGATCCAGCTT -3′; LKB1 Reverse: 5′- ACGTAGGCTGTGCAACCTCT -3′; three primers for the CNP-Cre PCR reaction: 5′- GCCTTCAAACTGTCCATCTC -3′; 5′- GATGGGGCTTACTCTTGC -3′ and 5′- CATAGCCTGAAGAACGAGA -3′. LKB1 primers amplify a 450-bp DNA fragment corresponding to the floxed allele and a 380-bp fragment corresponding to the wild-type allele. Three CNP-Cre primers generate a DNA fragment of 894 bp corresponding to the CNP-Cre allele and a 1,160-bp fragment for wild-type allele. Primary SC and DRG coculture Purified DRG and SC cultures were established using methods described previously (Lewallen et al . [13] ; Chan et al . [8] ). DRGs were removed from E15 rat embryos and placed in a 15-ml conical centrifuge tube with 5 ml of L15 medium+10% fetal bovine serum (FBS) and allowed to settle. The DRGs were washed with 10 ml of L15 medium and replaced with 5 ml of 0.25% trypsin. DRGs were then incubated at 37 °C for 45 min. Trypsin was removed and DRGs were washed by adding 10 ml of L15+10% FBS and centrifuged gently at 1,000 r.p.m. for 10 min. The medium was replaced with 5 ml of DRG medium containing high-glucose MEM, 10% FBS and 100 ng ml −1 NGF. Trituration was performed with a fire-polished Pasteur pipette until the suspension was homogeneous. The dissociated DRGs were plated on collagen-coated glass coverslips at a volume of 400 μl at a density of 150,000 total cells per 25-mm coverslip. The next day, the wells were flooded with 1 ml of medium containing antimitotic (high-glucose MEM, N2 supplement, 100 ng ml −1 NGF and FdU). After 2 days, the medium was replaced with 1 ml of DRG medium. The feeding cycle alternating between DRG medium and medium containing antimitotic was then repeated twice. The purified DRG neurons were cultured in DRG medium for an additional week before adding purified SCs. Two-day-old rat pups were used for SC isolation and purification from sciatic nerves. Nerves were placed in L15+10% FBS and allowed to settle. The nerves were washed with L15 then incubated at 37 °C for 15 min in 3 ml of 3 mg ml −1 collagenase solution. The collagenase was removed and replaced with fresh 3 ml collagenase solution with 500 μl of 0.25% trypsin for an additional incubation at 37 °C for 15 min. The collagenase solution was removed. The nerves were triturated with a fire-polished Pasteur pipette in 5 ml of L15+10% FBS until thoroughly teased. The suspension was filtered through a 40-μm cell strainer. The strainer was rinsed with 5 ml L15+10% FBS. The suspension was centrifuged at 1,500 r,p,m, for 15 min and cells were resuspended and cultured in SC medium (DMEM, 10% FBS and penicillin/streptomycin) on PLL-coated dishes. Cytosine arabinoside was added the next day at a final concentration of 1 mM. SCs were cultured for three more days before removal of cytosine arabinoside. The SC medium was replaced every 3 days and SCs were cultured for an additional week. Approximately 100,000 SCs were seeded on purified neurons and allowed to proliferate and ensheath the axons for ~5–7 days. Myelination was then initiated with the addition of ascorbic acid (50 μg ml −1 ). Dissociated SC/DRG coculture explants Dissociated SC/DRG cocultures were established using methods described previously [8] , [13] . DRGs were isolated from mouse embryos (E13–E14) and washed with L15 medium before incubation in 0.25% trypsin at 37 °C for 30 min. Trypsin was removed and DRGs were washed with L15+10% FBS and centrifuged gently at 1,000 r.p.m. for 10 min. The medium was replaced with DRG medium containing high-glucose MEM, 10% FBS and 100 ng ml −1 NGF. The ganglia were triturated with a fire-polished Pasteur pipette until the suspension was homogeneous and the dissociated DRGs were plated on collagen-coated glass coverslips at a density of ~150,000 cells per 25-mm coverslip. The cells were cultured in DRG medium for 5 days before ascorbic acid was added to induce myelination. CAP recordings Mice were anaesthetized with isofluorane, and sciatic nerves were isolated and transferred to oxygenated recording solution (125 mM NaCl, 2.5 mM KCl, 1 mM MgCl 2 , 2 mM CaCl 2 , 10 mM D -glucose, 1.25 mM NaH 2 PO 4 , 25 mM NaHCO 3 ) at room temperature. Both ends of the sciatic nerve were suctioned into separate fire-polished borosilicate glass suction electrodes using 2 ml precision syringes (Gilmont). A transparent adhesive grid slide with 1-mm spacing (Election Microscopy Sciences) was fixed underneath the recording chamber to measure the length of nerves (between suction electrodes). Signals were acquired with a differential AC amplifier (Model 1700, AM Systems) and digitized (Axon Digidata 1440A, Molecular Devices). Constant current stimulation (50 μs) was delivered to the stimulus electrode using a stimulus isolator (ISO-Flex, A.M.P.I.). Oxygenated recording solution was perfused by gravity into the recording chamber and removed via a peristaltic pump. CAPs were measured at room temperature by delivering current via the stimulus electrode on one end of the nerve, while recording the voltage response at the other end. Conductance velocity was determined by dividing the length of the nerve over the latency between the start of the stimulus artifact and the peak of the CAP. For paired stimulation experiments, the amplitude of the CAP was taken from a baseline immediately before the stimulus artifact and measured at the maximum positive voltage deflection during the CAP. Where the amplitude of the second CAP was too small to be identified by the eye, we measured the amplitude at a latency equal to that of the first CAP. Retroviral vectors The pCAG-IRES-EGFP-WT LKB1 and the S431A phospho-mutant constructs were obtained from Drs Mu-ming Poo and Maya Shelly. A NotI restriction site was engineered into 3′ region downstream of the coding sequence of LKB1 using PCR. The PCR products and the retroviral vector pBMN-I-GFP (Addgene) were digested with NotI. The digested PCR products were ligated into the viral vector and the constructs (pBMN-WT-LKB1-GFP and pBMN-S431A-LKB1-GFP) were confirmed by sequencing. pCAG-Cre and pBMN-I-GFP were digested with both EcoRI and NotI, respectively. The Cre fragment from pCAG-Cre was then ligated into the retroviral vector (pBMN-Cre-GFP). Retroviral production was achieved by transfecting Phoenix cells as previously described (Lewallen et al . [13] ). Viral supernatant was harvested 48–72 h post transfection and centrifuged to remove cellular debris. The retroviral supernatants were prepared in MEM medium containing 10% FBS and NGF and added to cocultures. Western blot analysis Samples from cultures and mouse sciatic nerves were prepared for western blot analysis as previously described [13] . Briefly, samples were dounced in RIPA buffer containing: 50 mM Tris, pH 8.0, 150 mM NaCl, 2 mM EDTA, 1 mM Na 3 VO 4 , 2.5 mM NaF, Complete protease inhibitor (Roche), 1% NP-40, 0.5% Na deoxycholic acid, 1 mM phenylmethylsulphonyl fluoride and 0.1% SDS for western blot analysis. Electrophoretic separation of the samples and the extracts was performed on 10% SDS polyacrylamide gels. Proteins were transferred to nitrocellulose membranes and probed with specific antibodies. Antibodies for western blot analysis were as follows: rat monoclonal anti-MBP (Millipore), mouse monoclonal anti-P0 (Astexx), mouse monoclonal anti-β-actin (Sigma), rabbit polyclonal anti-Oct-6 (provided by Dr Dies Meijer), rabbit polyclonal anti-Oct-6 (provided by Dr Dies Meijer), mouse monoclonal anti-LKB1 (Abcam), mouse monoclonal anti-p-LKB1 (Santa Cruz Biotechnology) and rabbit polyclonal anti- p75 NTR (Promega). The Alexa Fluor goat anti-rabbit, anti-mouse and anti-rat 680 IgG antibodies (Invitrogen) were used as secondary antibodies for near-infrared fluorescent detection performed on the Odyssey Infrared Imaging System (LI-COR). Full western blots from all the figures are displayed in Supplementary Fig. 3 . Immunostaining Immunostaining was performed as previously described [13] . Briefly, SC and SC-DRG cocultures were fixed using 4% paraformaldehyde, dehydrated and permeabilized and blocked by incubation with 20% goat serum and 0.2% Triton X-100 in PBS. Myelin was detected with a rat monoclonal anti-MBP antibody (Millipore, 1:100 dilution). Axons were detected using a rabbit polyclonal anti-neurofilament antibody (145 kDa, medium chain; Millipore, 1:200 dilution) and a mouse monoclonal anti-neurofilament antibody (Covance, 1:200 dilution). SCs were detected by using a rabbit polyclonal antibody to S100 (Dako, 1:500 dilution), rabbit polyclonal antibodies to Krox20 and Oct-6 (provided by Dies Meijer, 1:500 dilution) and a rabbit polyclonal antibody to Sox2 (provided by Samuel Pleasure, 1:100 dilution). Par-3 was detected using a rabbit polyclonal anti-Par-3 antibody (Provided by Dr Tony Pawson, 1:200 dilution). LKB1 was detected by using a mouse monoclonal anti-LKB1 antibody (Abcam, 1:50 dilution), rabbit polyclonal anti-LKB1 antibody (Abcam, 1:50 dilution), mouse monoclonal anti-phospho-S431-LKB1 antibody (Santa Cruz Biotechnology, 1:50 dilution) and rabbit polyclonal anti-phospho-S431-LKB1 antibody (Santa Cruz Biotechnology, 1:50 dilution). P75 NTR was detected using a rabbit polyclonal anti-p75 NTR antibody (Promega, 1:500 dilution). The Alexa Fluor anti-rat 594, anti-rabbit 488 and 594, and anti-mouse 488 and 594 IgG antibodies (Invitrogen, 1:1,000 dilution) were used as secondary antibodies for fluorescence detection. Cell nuclei were stained with mounting medium containing DAPI (Vectashield, Vector Labs). Co-localization was determined by fluorescence microscopy combined with Z-stack acquisition and 3D reconstruction performed on the Zeiss Apotome. Histology Animals were anaesthetized and perfused transcardially with PBS briefly, followed by 4% paraformaldehyde (Electron Microscopy Sciences). Sciatic nerves were removed and postfixed in 4% PFA overnight. Nerves were then submerged in 30% sucrose in PBS overnight. Sections that were 25-μm thick were obtained using a Microtome before immunostaining. Electron microscope analysis As previously described [13] , sciatic nerves were fixed through perfusion with 4% paraformaldehyde, and then submerged in 4% paraformaldehyde overnight. All nerves were stained with 1% osmium tetroxide for 1 h at 4 °C, and counterstained with 1% uranyl acetate overnight. Nerves were rinsed with distilled water and dehydrated in a series of ethanol dehydration treatments (50, 70, 95 and 100%). Embedding was performed in a 1:1 resin (EMBed-812, Electron Microscopy Services) and propylene oxide (Electron Microscopy Services) mix for 1 h at room temperature, followed by a 2:1 resin:propylene oxide mixture overnight at room temperature. Nerves were then placed in 100% resin for 3 h at room temperature. Ultrathin sections (70 nm) were obtained from the Norris Center Cell and Tissue Imaging Core at the University of Southern California, Keck School of Medicine and visualized with a JEM1400 Electron Microscope (JEOL) in the Zilkha Neurogenetic Institute. How to cite this article: Shen, Y.-A. A. et al . Phosphorylation of LKB1/Par-4 establishes Schwann cell polarity to initiate and control myelin extent. Nat. Commun. 5:4991 doi: 10.1038/ncomms5991 (2014).